Ultra-precise insertion of functional monomers in chain-growth polymerizations Chain-growth polymerizations are popular methods because they allow synthesis of high-molecular weight polymers in high yields and in short times. However, copolymers prepared by such processes generally exhibit uncontrolled monomer sequences. The controlled radical copolymerization of styrene with N -substituted maleimides is an interesting exception allowing preparation of controlled primary structures. However, because of the statistical nature of chain-growth mechanisms, sequence deviations are still present in these copolymers. Here we describe a specific range of experimental conditions that allows ultra-precise incorporation of a single N -substituted maleimide unit in a polystyrene chain. This occurs in a given kinetic regime where the styrene/ N -substituted maleimide comonomer ratio is very low. This situation usually only arises in the later stages of a chain-growth polymerization. Nevertheless, we show that it is possible to restore these particular kinetic conditions multiple times during a single polymerization by using successive feeds of donor and acceptor comonomers. For approximately 80 years, synthetic polymers have been prepared using two main mechanisms: chain-growth and step-growth polymerizations [1] . These two approaches allow synthesis of high-molecular weight macromolecules in relatively short times and are therefore used for the large-scale production of commodity plastics, as well as for the preparation of advanced functional materials such as conducting polymers [2] , biodegradable polymers [3] , shape-memory polymers [4] and malleable networks [5] . However, polymers synthesized via these mechanisms are not molecularly defined, but exhibit molecular weight and compositional distributions. This situation was significantly improved in recent decades, notably with the discovery of living and controlled chain-growth polymerizations [6] , [7] , [8] , [9] , [10] , [11] , [12] , which allow a better control over molecular parameters, such as chain length, functionality and topology [13] , [14] , [15] . Still, when two or more monomers are used in chain-growth or step-growth processes, polymers with poorly controlled comonomer sequence distributions are generally obtained [16] . This differs from the situation found in biopolymers, such as nucleic acids or proteins, in which each monomer unit is located at a precise position [17] . Sequence-defined oligomers and polymers can be synthesized using solid-phase chemistry [18] or biological concepts [19] , [20] , [21] . Dendrimer synthesis also allows a certain degree of control over molecular positioning [22] . However, precise sequence regulation is still not attained in chain-growth and step-growth polymerizations. Here we report an unprecedented level of molecular accuracy for the incorporation of functional monomers during a chain-growth polymerization. It was recently demonstrated that the controlled radical copolymerization of minute amounts of acceptor monomers (for example, maleic anhydride or N -substituted maleimides) in the presence of large excess of a donor monomer (for example, styrene) allows synthesis of polymers with controlled sequence distributions [23] , [24] . This behaviour is a consequence of the highly pronounced copolymerization tendency of donor/acceptor comonomer pairs combined with a living chain-growth mechanism [25] . However, even in such kinetically favourable conditions, statistical events are inevitable and result in local chain-composition uncertainties. In the present work, these deviations are reduced to a minimum approaching ideal mono-insertion conditions. Using kinetically controlled sequential additions of donor and acceptor monomer feeds, ultra-narrow insertion was obtained. It was demonstrated that this simple procedure allows precise molecular placement of functional monomers at virtually any chain location. Identification of the ultra-precise insertion conditions Because of the opposite polarity of their double bonds, donor (A) and acceptor (B) monomers have a very strong tendency to copolymerize in radical chain-growth polymerizations [26] . This feature is often exploited to synthesize alternating copolymers with regular monomer sequences ABABAB, using equimolar or near-equimolar feeds of comonomers. If a non-equimolar feed mixture is used (for example, large excess of donor as compared with acceptor), AB alternation is occurring in the early stages of the reaction, followed by homopolymerization of the excess of donor [25] . When combined with a controlled/'living' chain-growth mechanism (that is, a kinetically controlled process, in which all polymer chains grow simultaneously at the same rate), the composition drift of a non-equimolar feed is engraved in the microstructure (that is, the sequence of monomers) of each chain formed in the reaction [23] , [24] , [27] . This unique feature was recently exploited by our group to design polymers with complex microstructures and topologies [24] , [28] , [29] , [30] . However, in such approaches, monomer sequences are controlled but are not perfectly ordered. Because of the uneven ratio between donor and acceptor monomers, a certain level of uncertainty is inherent to these strategies ( Fig. 1 ). In fact, the higher the donor/acceptor ratio, the broader the sequence distribution. This particular aspect is illustrated by a series of model experiments ( Supplementary Table S1 and Fig. 2 ) and by the related microstructures shown in Fig. 1 . In these experiments, a minute amount of N -propyl maleimide (Pr-MI, 1 Eq.) was added at different stages of the nitroxide-mediated polymerization (NMP) of a large excess of styrene (50 Eq.). NMP is a controlled/'living' radical polymerization method that provides precise kinetic control of donor/acceptor copolymerizations [8] , [23] . When Pr-MI is added at the beginning of the reaction together with styrene ( Fig. 1a ), kinetic monitoring of comonomer conversion shows that it is incorporated in the growing chains at the early phase of the polymerization process, however, in a relatively broad statistical region. Typically, the Pr-MI unit is located somewhere in a zone of uncertainty containing about 10 styrene units in average. If Pr-MI is added later in the process, for example at half styrene conversion as schematized in Fig. 1b , the donor/acceptor ratio is lower than in the previous case and therefore a narrow statistical region is created (that is, the zone of uncertainty is restricted to about 5 styrene units in average). Very interestingly, when Pr-MI is added at high styrene conversion ( Fig. 1c ), statistical uncertainty starts to be considerably minimized. Indeed, at this stage of the reaction, the complete chain incorporation of a single Pr-MI unit is accompanied by only 1 or 2 styrene units in average. This suggests the formation of local regions with a controlled composition A/B 2:1. Such regions may indeed be constituted of different triads, that is, ABA, AAB or BAA. It has been reported that 13 C nuclear magnetic resonance (NMR) can be used to quantify triads of donor/acceptor copolymers [31] . However, in the present case, the molar fraction of the N -substituted maleimides in the formed copolymer chains is too low to allow reliable visualization of these triads, even using high-field NMR. Still, the kinetic data clearly indicate that the formed regions contain a near-perfect amount of donor and acceptor comonomers. At the extreme case, when the acceptor comonomer is added after styrene homopolymerization (that is, in the absence of styrene as shown in Fig. 1d ), chain-end mono-functionalization is attained, as elegantly demonstrated by Hawker and coworkers [32] . Yet, in these extreme conditions, the living character of the reaction is rapidly lost due to kinetically favored side reactions. 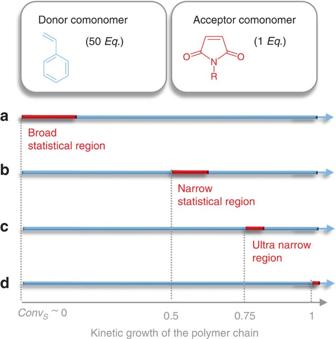Figure 1: General concept. Strategy studied for the synthesis of sequence-regulated polymers by controlled/'living' radical copolymerization of a large excess of a donor monomer (styrene) and an acceptor comonomer (N-substituted maleimide). Depending on the time of addition of the acceptor comonomer during the copolymerization, microstructures containing broad statistical region (a), narrow statistical region (b), ultra-narrow controlled region (c) or defined chain ends (d) can be obtained. Figure 1: General concept. Strategy studied for the synthesis of sequence-regulated polymers by controlled/'living' radical copolymerization of a large excess of a donor monomer (styrene) and an acceptor comonomer ( N -substituted maleimide). Depending on the time of addition of the acceptor comonomer during the copolymerization, microstructures containing broad statistical region ( a ), narrow statistical region ( b ), ultra-narrow controlled region ( c ) or defined chain ends ( d ) can be obtained. 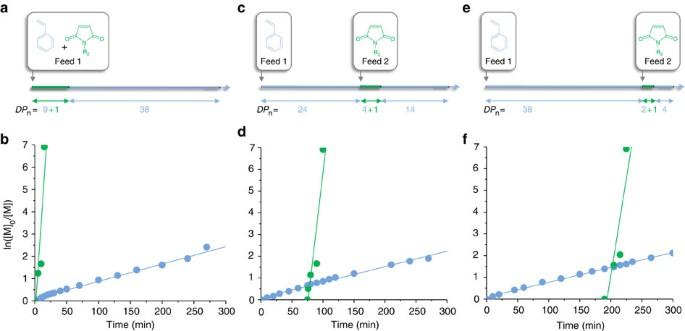Figure 2: Synthesis of model sequence-controlled polymers by NMP of styrene and Pr-MI. (a) Probable microstructure obtained when Pr-MI (R2=propyl) was added at the beginning of the experiment (P1 inSupplementary Table S1). Blue and green colours denote styrene and Pr-MI, respectively. (b) Semilogarithmic plots of monomer conversion versus time recorded for P1. (c) Probable microstructure obtained when Pr-MI was added at half styrene conversion (P2 inSupplementary Table S1). (d) Semilogarithmic plots of monomer conversion versus time recorded for P2. (e) Probable microstructure obtained when Pr-MI was added at 75% styrene conversion (P3 inSupplementary Table S1). (f) Semilogarithmic plots of monomer conversion versus time recorded for P3. Full size image Figure 2: Synthesis of model sequence-controlled polymers by NMP of styrene and Pr-MI. ( a ) Probable microstructure obtained when Pr-MI (R 2 =propyl) was added at the beginning of the experiment (P1 in Supplementary Table S1 ). Blue and green colours denote styrene and Pr-MI, respectively. ( b ) Semilogarithmic plots of monomer conversion versus time recorded for P1. ( c ) Probable microstructure obtained when Pr-MI was added at half styrene conversion (P2 in Supplementary Table S1 ). ( d ) Semilogarithmic plots of monomer conversion versus time recorded for P2. ( e ) Probable microstructure obtained when Pr-MI was added at 75% styrene conversion (P3 in Supplementary Table S1 ). ( f ) Semilogarithmic plots of monomer conversion versus time recorded for P3. Full size image Experimental validation of the ultra-precise concept The situation displayed in Fig. 1c was the starting point of the present work. The possibility of forming AB ordered sequences on short-chain sections is indeed an unusual, thus remarkable, feature for a chain-growth polymerization. It should be noted, however, that two types of deviations exist in these syntheses. Besides the uncertainty of positioning described in the previous paragraph, chain-to-chain composition drifts also exist. Matrix-assisted laser desorption/ionization–time of flight mass spectroscopy analysis of a short model polymer ( Supplementary Tables S2 and S7 and Supplementary Fig. S1 ) was used to study the latter aspect. This measurement suggested that polymers, synthesized in the conditions highlighted in Fig. 1c , exhibit very narrow composition distributions. Altogether, the model studies account for the 'ultra-precise' insertion of the N -substituted maleimide in the polystyrene chains. However, the situation shown in Fig. 1c is limited to a narrow range of styrene conversion, typically to values >60%. Here we demonstrate that this unique kinetic situation can be restored multiple times in a single polymerization and therefore used for repeated insertion of various functional N -substituted maleimides. This can be achieved under carefully optimized donor monomer-starved conditions. Instead of adding the whole quantity of donor monomer at the beginning of the reaction (that is, conventional approach), small successive feeds of donor and acceptor were used. The main advantage of this strategy is that it constantly preserves a low donor/acceptor ratio in the polymerization medium, and thus ultra-narrow insertion conditions. In order to demonstrate its versatility, this strategy was tested in three different types of controlled radical chain-growth polymerizations, namely NMP, activators regenerated by electron transfer for atom transfer radical polymerization (ARGET ATRP) and single-electron transfer living radical polymerization (SET-LRP) [33] , [34] . The latter two methods belong to a 'second generation' of controlled radical polymerizations, which allow an extremely fine control over macromolecular structure together with a minimal loss of active chain ends [35] , [36] . 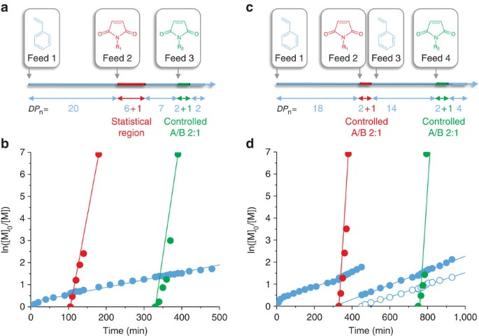Figure 3: Conventional and ultra-precise synthesis of sequence-controlled polymers containing two different MIs by ARGET ATRP. (a) Probable microstructure of the polymer prepared via a conventional three-step strategy (P10 inSupplementary Table S4). Blue, red and green colours denote styrene, Bz-MI (R1=benzyl) and Pr-MI (R2=propyl), respectively. (b) Semilogarithmic plots of monomer conversion versus time recorded for the conventional strategy. (c) Probable microstructure of the polymer prepared via a four-step ultra-precise strategy (P11 inSupplementary Table S4). (d) Semilogarithmic plots of monomer conversion versus time recorded for the ultra-precise strategy. For styrene, the full symbols denote the overall conversion, whereas the open symbols represent the conversion occurring after feed 3. Figure 3 compares the results of the conventional and ultra-precise approaches for ARGET ATRP polymerizations, in which two functional N -substituted maleimides were added. In both experiments, similar chain lengths and microstructures were targeted. In the conventional approach ( Fig. 3a,b ), the whole amount of styrene was added at the beginning of the reaction (feed 1, 45 Eq.) followed by two successive additions of the acceptor comonomers (feeds 2 and 3, 1 Eq. each). As demonstrated in previous publications [24] , [25] , this method allowed local positioning of the N -substituted maleimides in the polystyrene chains. However, a detailed analysis of the copolymerization kinetics confirmed that the first N -substituted maleimide is incorporated in broad statistical region. In comparison, the ultra-precise strategy led to much more precise microstructures ( Fig. 3c,d ). In this approach, styrene homopolymerization was first started with a small batch of styrene (feed 1, 25 Eq.). When styrene conversion reached the suitable range for ultra-narrow insertion (that is, 70% in this particular case), N -benzyl maleimide (Bz-MI) was added in the reaction medium (feed 2, 1 Eq.). 1 H NMR monitoring of the copolymerization kinetics confirmed the ultra-precise insertion of Bz-MI in the chains. Indeed, 50 min after feed 2, the conversion of Bz-MI was above 99% (that is, 1 unit of Bz-MI was added in average in each polymer chain), whereas styrene conversion gained 7% only (that is, 2 styrene units were added in average in each polymer chain). These numbers suggest a precise A/B 2:1 alternation in this portion of the formed chains. Shortly after the full consumption of Bz-MI, a second batch of styrene (feed 3, 20 Eq.) was added in the polymerization medium in order to refresh chain growth. This new batch completed the residual styrene, which was not polymerized during the first phase of the reaction (that is, about 4 Eq.). The semilogarithmic plots of comonomer conversion versus time ( Fig. 3d ) and the evolution of the size-exclusion chromatography (SEC) versus time ( Fig. 4 ) indicated that chain-growth polymerization continued to proceed in a controlled/'living' fashion after feed 3. When styrene conversion reached again the proper range for ultra-precise addition, Pr-MI was added in the medium (feed 4, 1 Eq.). Copolymerization kinetics confirmed the ultra-narrow insertion of this second N -substituted maleimide. Afterwards, styrene homopolymerization was pursued for a short time until the experiment was stopped. SEC ( Supplementary Table S6 ) and 1 H NMR analysis of the final purified polymer confirmed the formation of a well-defined structure with a narrow molecular weight distribution (monomodal SEC chromatograms), controlled molecular weight and exact comonomer composition. These results obtained by ARGET ATRP confirm that the ultra-precise strategy is viable and allows construction of complex microstructures with precise functional regions. Comparable results were also obtained in NMP ( Supplementary Table S3 and Supplementary Fig. S2 ) and SET-LRP ( Supplementary Table S5 and Supplementary Fig. S3 ) experiments. However, in NMP experiments, it was observed that experimental M n values closely matched theoretical predictions during the first regime of the experiment (that is, after feed 1) but became higher than theory after the second addition of styrene (that is, after feed 3). Figure 3: Conventional and ultra-precise synthesis of sequence-controlled polymers containing two different MIs by ARGET ATRP. ( a ) Probable microstructure of the polymer prepared via a conventional three-step strategy (P10 in Supplementary Table S4 ). Blue, red and green colours denote styrene, Bz-MI (R 1 =benzyl) and Pr-MI (R 2 =propyl), respectively. ( b ) Semilogarithmic plots of monomer conversion versus time recorded for the conventional strategy. ( c ) Probable microstructure of the polymer prepared via a four-step ultra-precise strategy (P11 in Supplementary Table S4 ). ( d ) Semilogarithmic plots of monomer conversion versus time recorded for the ultra-precise strategy. For styrene, the full symbols denote the overall conversion, whereas the open symbols represent the conversion occurring after feed 3. 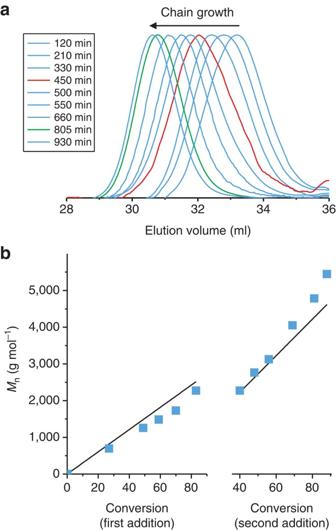Figure 4: Molecular weight control in the ARGET ATRP ultra-precise strategy. (a) SEC chromatograms recorded in THF at different stages of the ultra-precise synthesis (P11 inSupplementary Table S4). The red and green colours indicate the incorporation of Bz-MI and Pr-MI during the chain-growth process. (b) Corresponding plots ofMnversus overall styrene conversion. Full size image Figure 4: Molecular weight control in the ARGET ATRP ultra-precise strategy. ( a ) SEC chromatograms recorded in THF at different stages of the ultra-precise synthesis (P11 in Supplementary Table S4 ). The red and green colours indicate the incorporation of Bz-MI and Pr-MI during the chain-growth process. ( b ) Corresponding plots of M n versus overall styrene conversion. Full size image Extension to the synthesis of tailored microstructures The ultra-precise strategy is not restricted to the chain length and microstructure shown in Fig. 3 and Supplementary Figs S2 and S3 . Both parameters can be easily varied by simply changing the amount and time of addition of each feed ( Fig. 5 ). As a consequence, the ultra-precise approach can be used to synthesize polymer chains containing N -substituted maleimides at any desired location. In addition, this strategy can be applied to the synthesis of more complex sequence-controlled polymers. For instance, Fig. 6 shows the synthesis by SET-LRP of copolymers containing three different N -substituted maleimides positioned in their chains. The conventional approach involving three successive feeds of acceptor monomers ( Fig. 6a ) led to statistical insertions for the first two monomers and to a narrower insertion for the last monomer only. On the other hand, an ultra-precise strategy involving six successive feeds of donor and acceptor comonomers ( Fig. 6b ) led to well-defined polymers containing precisely positioned N -substituted maleimides. 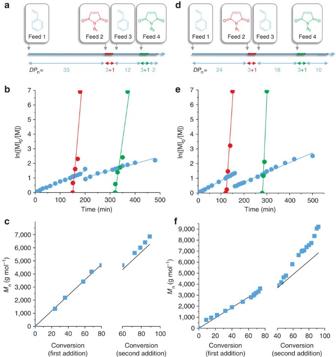Figure 5: Synthesis of polymers with different microstructures using a four-feed ultra-precise strategy in NMP. (a) Synthesis of copolymer with precise incorporation of Bz-MI (R1=benzyl) and Pr-MI (R2=propyl) at 2/3 of the chain length and close to the ω-chain-end, respectively (P8 inSupplementary Table S3). (b) Semilogarithmic plots of monomer conversion versus time for P8. Blue, red and green colours denote styrene, Bz-MI and Pr-MI, respectively. (c) Plots ofMnversus overall styrene conversion for P8. (d) Synthesis of copolymer with precise incorporation of Bz-MI and Pr-MI at 2/5 and 3/4 of the chain-length, respectively (P9 inSupplementary Table S3). (e) Semilogarithmic plots of monomer conversion versus time for P9. (f) Plots ofMnversus overall styrene conversion for P9. Figure 5: Synthesis of polymers with different microstructures using a four-feed ultra-precise strategy in NMP. ( a ) Synthesis of copolymer with precise incorporation of Bz-MI (R 1 =benzyl) and Pr-MI (R 2 =propyl) at 2/3 of the chain length and close to the ω-chain-end, respectively (P8 in Supplementary Table S3 ). ( b ) Semilogarithmic plots of monomer conversion versus time for P8. Blue, red and green colours denote styrene, Bz-MI and Pr-MI, respectively. ( c ) Plots of M n versus overall styrene conversion for P8. ( d ) Synthesis of copolymer with precise incorporation of Bz-MI and Pr-MI at 2/5 and 3/4 of the chain-length, respectively (P9 in Supplementary Table S3 ). ( e ) Semilogarithmic plots of monomer conversion versus time for P9. ( f ) Plots of M n versus overall styrene conversion for P9. 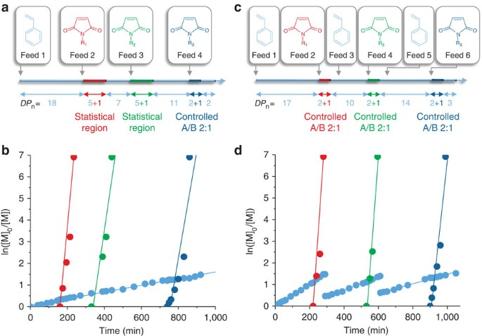Figure 6: Conventional and ultra-precise synthesis of sequence-controlled polymers containing three different MIs by SET-LRP. (a) Probable microstructure of the polymer prepared via a conventional four-step strategy (P13 inSupplementary Table S5). Blue, red, green and dark blue colours denote styrene, Bz-MI (R1=benzyl), Pr-MI (R2=propyl) and PFP-MI (R3=pentafluorophenyl benzoate) respectively. (b) Semilogarithmic plots of monomer conversion versus time recorded for the conventional strategy. (c) Probable microstructure of the polymer prepared via a six-step ultra-precise strategy (P15 inSupplementary Table S5). (d) Semilogarithmic plots of monomer conversion versus time recorded for the ultra-precise strategy. Full size image Figure 6: Conventional and ultra-precise synthesis of sequence-controlled polymers containing three different MIs by SET-LRP. ( a ) Probable microstructure of the polymer prepared via a conventional four-step strategy (P13 in Supplementary Table S5 ). Blue, red, green and dark blue colours denote styrene, Bz-MI (R 1 =benzyl), Pr-MI (R 2 =propyl) and PFP-MI (R 3 =pentafluorophenyl benzoate) respectively. ( b ) Semilogarithmic plots of monomer conversion versus time recorded for the conventional strategy. ( c ) Probable microstructure of the polymer prepared via a six-step ultra-precise strategy (P15 in Supplementary Table S5 ). ( d ) Semilogarithmic plots of monomer conversion versus time recorded for the ultra-precise strategy. Full size image The controlled radical chain-growth copolymerization of styrene with various N -substituted maleimides was studied. These experiments were performed in non-stoichiometric conditions using an excess of donor monomer and time-controlled additions of minute amounts of the acceptor comonomers. We have identified a specific range of experimental conditions that allows a highly precise insertion of a single N -substituted maleimide unit in the copolymer chains. This occurs in a particular kinetic regime where the donor/acceptor comonomer ratio is very low. This situation usually happens at the end of the copolymerization when the donor monomer is significantly consumed. However, it is possible to restore these kinetic conditions multiple times during the same polymerization by using consecutive feeds of donor and acceptor comonomers. As a consequence, functional acceptor comonomers can be positioned at very precise chain locations. Such precision for controlling the microstructure of polymers in a radical chain-growth process is unprecedented. The strategy is experimentally easy and can be applied in various types of controlled radical chain-growth polymerizations. For instance, in the present work, this new concept was successfully tested in NMP, ARGET ATRP and SET-LRP. However, the three methods did not provide the same quality of results. In NMP experiments, it was observed that experimental M n became significantly higher than theory after applying the ultra-precise strategy. This trend was also observed in SET-LRP and ARGET ATRP experiments, but to a lesser extent. In fact, it should be pointed out that the high conversion regime, required for the ultra-precise strategy, may also favour side reactions, such as termination and eliminations [37] . Hence, our concept implies that the reaction should be 'revitalized' by adding fresh styrene before losing significantly the living character of the reaction. The experimental data show that it is possible in SET-LRP and ARGET ATRP but more critical in NMP. Models of homopolymer studies ( Supplementary Fig. S4 ) indicated that this behaviour is not a consequence of the addition of the N -substituted maleimide (for example, due to elimination occurring on this particular monomer unit). Indeed, similar plots of M n versus conversion were observed for homopolymerizations employing two successive styrene feeds. This implies that the observed deviations are due to termination reactions inherent to the NMP mechanism, as suggested by the high molecular-weight shoulder and low molecular-weight tailing in the final NMP chromatograms. It was also evidenced that the ultra-precise concept is versatile. Indeed, the functional N -substituted maleimides can be placed virtually anywhere in the copolymer chains. Moreover, the experimental results show that up to three different N -substituted maleimides can be incorporated in the chains using this approach. However, in such a case, it seems mandatory to use controlled radical polymerization techniques with a very high degree of control, such as SET-LRP and ARGET ATRP. It should be also clearly specified that the ultra-precise strategy can probably not be repeated indefinitely. As mentioned above, side reactions occur in radical chain-growth polymerizations, and at some point, the living character of the reaction will be inevitably lost. Nevertheless, in proper experimental conditions, tailor-made polymeric microstructures are attainable using this approach. Moreover, the ultra-precise strategy is not restricted to the model monomers employed here and can be potentially extended to a very broad range of monomers. First of all, a large number of N -substituted maleimides can be used in sequence-controlled copolymerizations. We have been developing so far a library of about 25 different entries [25] . For example, N -substituted maleimides bearing reactive groups, hydrophilic functions, fluorophores, bio-recognition moieties and stimuli-responsive functions can be utilized. In addition, it is also possible to vary the nature of the donor monomer. Styrene can be, for example, replaced by functionally substituted styrenics. Thus, the main properties of the polymer chain can also be tuned. For instance, sequence-controlled water-soluble polymers can be prepared [38] , [39] . Overall, the present results open a wide spectrum of opportunities in synthetic polymer science. Materials BlocBuilder MA, (Arkema, 97%), N -benzylmaleimide (Alfa Aesar, 99%), N -(n-propyl)maleimide (Alfa Aesar, 94%), anisole (Sigma Aldrich, 99%), toluene (Sigma Aldrich, ≥99.7% puriss. stabilized), methanol (Carlo Erba, 99.9%), tetrahydrofuran for SEC (Sigma Aldrich, 99.8% HPLC, stabilizer-free), N , N , N ′, N ″, N ″-pentamethyldiethylenetriamine (Sigma Aldrich, 99%), CuBr (Sigma Aldrich, 98%), copper powder (Alfa Aesar, 99.5%), CuBr 2 (Alfa Aesar, 99%), ethyl 2-bromopropionate (Sigma Aldrich, 99%), methyl 2-bromopropionate (Sigma Aldrich, 99%), tin(II) 2-ethylhexanoate (Sn(EH) 2 , Alfa Aesar, 96%) and tris(2-dimethylaminoethyl)amine (Me 6 TREN, Alfa Aesar, 99+%) were used as received. Styrene (Sigma Aldrich, >99%) was distilled over CaH 2 (90–95%) under reduced pressure and stored under an argon atmosphere at −15 °C. Tetrahydrofurane (THF, >99.9%, reagent grade, stabilized with butylated hydroxytoluene) was distilled from sodium benzophenone before use. The synthesis of pentafluorophenyl 4-maleimidobenzoate (PFP-MI) was described in a previous publication [40] . General polymerization procedures Three different types of controlled radical chain-growth polymerizations, NMP, ARGET ATRP and SET-LRP, were used for the synthesis of polymers with controlled microstructure. The NMP of styrene was carried out as follows: the monomer (different targeted DP n ), anisole (1:1 volume ratio with respect to styrene) and commercially available alkoxyamine BlocBuilder MA were weighted in a Schlenk tube. The sealed tube was degassed with dry argon and then immersed in a preheated oil bath thermostated at 120 °C for several hours. The ARGET ATRP of styrene was adapted from the literature [35] and was undertaken as follows: a deoxygenated solution of CuBr and Me 6 TREN as ligand was prepared in a Schlenk tube with the appropriate amounts of degassed styrene, Sn(EH) 2 as reducing agent and degassed toluene as solvent (1:1 volume ratio with respect to styrene). The degassed Schlenk tube was placed into a thermostated oil bath at 110 °C for several hours, after addition of a known volume of methyl 2-bromopropionate as initiator. The SET-LRP procedure was adapted from the literature [36] . Copper powder, CuBr 2 , degassed monomer (different targeted DP n ), degassed toluene (1:2 volume ratio with respect to styrene), N,N,N ′ ,N″ , N″ -pentamethyldiethylenetriamine and lastly ethyl 2-bromopropionate were added into a Schlenk tube. The tube was sealed, degassed with dry argon and subsequently heated at 90 °C in an oil bath for several hours. Conventional sequence-controlled strategy In these procedures, the whole amount of styrene was added at the beginning of reaction in one feed, as described in the previous paragraph. For NMP and ARGET ATRP, small amounts of N -benzylmaleimide and/or Pr-MI previously dissolved in the corresponding solvent were successively added in the polymerization mixture, at different stages of the reactions, using degassed syringes. For SET-LRP process, a third MI was successively incorporated in the polymer chains, namely PFP-MI. Additional details about the time-controlled addition of the N -substituted maleimides can be found in the Supplementary Methods. Samples were withdrawn periodically from the polymerization mixtures and analysed by SEC and 1 H NMR to determine molecular weights and the incorporation of N -substituted maleimides in the growing polymer chains, respectively. Ultra-precise sequence-controlled strategy In this approach, NMP, ARGET ATRP or SET-LRP of styrene is first started using a small batch of monomer. After a given time, when styrene conversion reached a value >60%, considered to be proper for the ultra-precise addition, N -benzylmaleimide dissolved in the corresponding solvent was injected in the reaction mixture using a degassed syringe. Just after the complete consumption of Bz-MI, a second batch of degassed styrene was introduced in the reaction medium completing the leftover amount of styrene from the first stage of reaction. When overall styrene conversion was again >60%, a solution of Pr-MI previously prepared and degassed was added in the medium. After the full incorporation of Pr-MI in the growing polymer chains, styrene homopolymerization was pursued until it reached conversions in the range of 88–96%. In some cases, a third batch of degassed styrene was introduced in the reaction mixture to complete the unreacted amount of monomer from the previous stages of reaction and the polymerization proceeded until 73% conversion. At this stage, a hot solution of PFP-MI in toluene was injected in the polymerization mixture in order to be incorporated in the growing polymer chains. After the complete consumption of PFP-MI, the polymerization was stopped. For all stages of the polymerization, samples were withdrawn periodically and analysed by SEC and 1 H NMR to determine molecular weights and the incorporation of N -substituted maleimides in the growing polymer chains respectively. All the polymerizations were stopped by exposing the reaction mixtures to air, dissolved in THF and the polymers precipitated in cold methanol. Measurements SEC measurements were performed on five PLgel 10 μ Mixed-B columns and using a Shimadzu SPD M20A refractive index detector. The mobile phase was THF with a flow rate of 1 ml min −1 using a Shimadzu LC20AD pump. Toluene was used as internal reference. The molecular-weight calibration was based on 16 narrow molecular-weight linear polystyrene standards from Polymer Laboratories. 1 H NMR spectra were recorded in CDCl 3 on a Bruker Avance 400 MHz spectrometer. Styrene conversion was calculated from the 1 H NMR spectra of the raw experimental samples by comparing the integration of two vinyl protons of remaining styrene at 5.69 and 5.18 ppm to the integration of the region 6.25–7.5 ppm, which contains five aromatic protons of the formed polymer and of unreacted monomer, one methine proton of the remaining styrene, five aromatic protons of the solvent (anisole for NMP or toluene for SET-LRP and ARGET ATRP) and at some stages of reaction 7 protons belonging to the added Bz-MI, five protons of the polymerized Bz-MI, six protons of the added PFP-MI, six protons of polymerized PFP-MI and two protons of the added Pr-MI. It should be noted that two different types of styrene conversion can be calculated in the ultra-precise experiments. Additional information about these calculations can be found in Supplementary Note 1 . The conversions of N -substituted maleimides were also estimated by 1 H NMR as follows: for Bz-MI, the evolution of the singlet at 4.6 ppm was monitored, whereas in case of Pr-MI, the triplet at 3.4 ppm (two methylene protons in alpha of the maleimide function) was analysed. Because of the overlapping of characteristic signals of the protons belonging to these two MIs, either with the specific signal of the proton in alpha of the bromide chain end (4.3 ppm) or with the signal of methyl protons of the initiator (MBP, 3.5 ppm), the conversion was appreciated with respect to the integration of the specific signal of methyl protons of toluene (2.27 ppm). For PFP-MI, the evolution of the doublet at 8.23 ppm (two aromatic protons in meta of the maleimide function) was monitored. Matrix-assisted laser desorption/ionization–time of flight mass spectra were acquired on a Bruker Daltonics Auto Flex system equipped with a 337-nm N 2 laser, in the positive ion and reflectron mode using polystyrene as a positive external standard. Dithranol was used as matrix (10 mg ml −1 in THF). Matrix, ionization agent (AgTFA) and polymer sample were mixed in a 10:1:2 ratio. A volume of 0.5 μl of the solution was applied on the target. How to cite this article: Zamfir, M. & Lutz, J.-F. Ultra-precise Insertion of functional monomers in chain-growth polymerizations. Nat. Commun. 3:1138 doi: 10.1038/ncomms2151 (2012).